Direct observation of prompt pre-thermal laser ion sheath acceleration High-intensity laser plasma-based ion accelerators provide unsurpassed field gradients in the megavolt-per-micrometer range. They represent promising candidates for next-generation applications such as ion beam cancer therapy in compact facilities. The weak scaling of maximum ion energies with the square-root of the laser intensity, established for large sub-picosecond class laser systems, motivates the search for more efficient acceleration processes. Here we demonstrate that for ultrashort (pulse duration ~30 fs) highly relativistic (intensity ~10 21 W cm −2 ) laser pulses, the intra-pulse phase of the proton acceleration process becomes relevant, yielding maximum energies of around 20 MeV. Prominent non-target-normal emission of energetic protons, reflecting an engineered asymmetry in the field distribution of promptly accelerated electrons, is used to identify this pre-thermal phase of the acceleration. The relevant timescale reveals the underlying physics leading to the near-linear intensity scaling observed for 100 TW class table-top laser systems. In recent years, target-normal-sheath-acceleration (TNSA) [1] has been established as a robust source of intense multi 10 MeV proton pulses for a wide range of laser and target parameters [2] , [3] , [4] , [5] . Protons originating from hydrogenated contaminants on the target surfaces gain initial energy in the electric field that arises when electrons, laser-heated to megaelectronvolt temperatures, are driven out of the solid target volume. This heating of electrons may take place at the critical density surface of the target front side, potentially modified by preplasma formation, or throughout the target volume when relativistic transparency sets in [6] , [7] . Generally, the field strength increases with electron density and the electron temperature in the thermal sheath. The plasma then expands [8] in longitudinal and transverse directions leading to a continuous decrease in electron density and temperature, while energy is transferred to the proton ensemble. For sufficiently long pulses (typically exceeding 100 fs), this mechanism is known to lead to exponential proton energy spectra, with a cutoff energy that scales with the square root of the laser intensity. Recent experiments have shown that a restriction of the target area may confine the electron sheath and allow for more efficient re-heating and thus increased proton energies [9] , [10] . Yet, such approaches are again limited to longer pulse durations matching such transverse electron recirculation timescales. As a consequence, the use of ultrashort pulses for reaching energies above 100 MeV seemed to be discouraging. The ongoing development of ultrashort pulse high-intensity Ti:sapphire-based laser systems into the multi-petawatt range has shifted the interest to timescales where the early phase of the TNSA plasma expansion model [8] has to be revisited. Within typical laser pulse durations of 30 fs, the motion of relativistic electrons is restricted to only several micrometer, and thus longitudinal recirculation. A significant transverse expansion or cooling can be neglected during the initial acceleration phase. The original hot-electron distribution, depending strongly on the governing laser absorption mechanism and likely to be anisotropic, and thus non-thermal, in a three-dimensional picture, will directly feed the accelerating field. Here we demonstrate that protons efficiently gain energy during this ultrashort initial period, the intra-pulse phase. Non-target-normal proton emission In the typical proton acceleration experiment, presented in Fig. 1 , the ultrashort laser pulse impinges under an angle of δ =45° onto a micron-thick solid target. Energetic protons are recorded behind the foil using a radiochromic film (RCF) stack, from which the spatial energy distribution can be reconstructed with large angle acceptance (see Methods ). Here a deflection of the most energetic protons, of about 5° from target normal into the direction of the initial laser propagation axis, is observed whereas lower energy protons exhibit a symmetric pattern with a larger divergence angle. In the following, this directed deflection of energetic protons will be correlated with the directed acceleration of hot electrons in the presence and thus on the timescale of the ultrashort laser pulse. 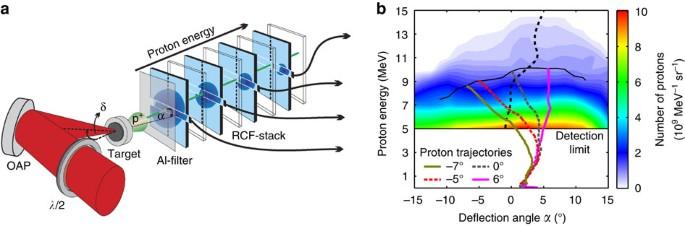Figure 1: Spatial energy distribution of laser-accelerated proton beams. (a) The accelerating laser pulse is tightly focussed by an off-axis parabolic mirror (OAP) under oblique incidence (δ=45°,p-polarization) onto a 2-μm thick titanium foil target, and proton emission is recorded with stacks (about 15 layers covered with aluminum) of RCF. In front of the off-axis parabola a half-wave plate (λ/2) can be inserted to change the laser polarization. The reconstruction of the particle number per energy for horizontal slices of the RCF dose distributions (seeMethods) indicated with the black arrows yields the angularly resolved proton energy spectrum shown in (b). The dashed black line represents the centroid of the angular distribution. Scaled trajectories for protons reaching 70% of the maximum energy (black solid line) at different final deflection angles (α) are added. Figure 1: Spatial energy distribution of laser-accelerated proton beams. ( a ) The accelerating laser pulse is tightly focussed by an off-axis parabolic mirror (OAP) under oblique incidence ( δ =45°, p -polarization) onto a 2-μm thick titanium foil target, and proton emission is recorded with stacks (about 15 layers covered with aluminum) of RCF. In front of the off-axis parabola a half-wave plate ( λ /2) can be inserted to change the laser polarization. The reconstruction of the particle number per energy for horizontal slices of the RCF dose distributions (see Methods ) indicated with the black arrows yields the angularly resolved proton energy spectrum shown in ( b ). The dashed black line represents the centroid of the angular distribution. Scaled trajectories for protons reaching 70% of the maximum energy (black solid line) at different final deflection angles ( α ) are added. Full size image For a time-resolved analysis of the interaction process, the 2D3 V particle in cell code PICLS [11] was applied. Target surface conditions were simulated self-consistently making use of measured temporal profiles of the laser pulse starting at t =−3.5 ps where ionization first sets in (see Methods ). 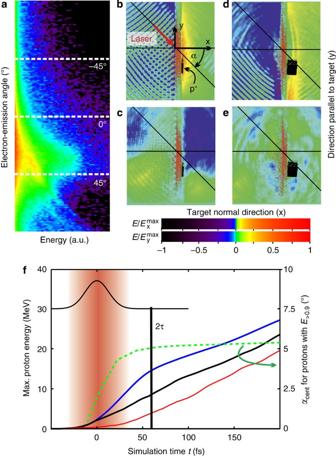Figure 2: Modelling the intra-pulse acceleration. (a) False-colour image (logarithmic scale) of the angularly resolved electron energy distribution at the target rear side, at the time the peak of the laser pulse reaches the front side (t=0). The components of the spatial distribution of the electric field amplitude in target normal direction (Ex), and parallel to the target surfaces (Ey), are plotted in (b) and (c) fort=0, and in (d) and (e) fort=44 fs, respectively. The field distributions are normalized using the maximum field values ofThe edge size of the boxes (b–e) corresponds to 18 μm. The trajectories of protons reaching more than 90% of the maximum energy (E>0.9) are overlaid in black. (f) For these protons, the increase of the deflection angleαcentwith time is shown in green, together with the evolution of the maximum energy of protons emitted under sample anglesαof 6° (blue), −1° (black) and −5° (red). For illustration of the timescale, the laser pulse profile is given by the red shaded region and the black gaussian-shaped curve. For the duration of the laser pulseτ, the asymmetry of the electron distribution translates into a non-target-normal emission of energetic protons that can be detected experimentally. Figure 2a shows a snapshot of the electron energy distribution, plotted as a function of the emission angle at the time the peak of the pulse reaches the target front side ( t =0; further time steps are given in Supplementary Fig. S1 ). Because of the pronounced correlation of the distribution with the direction of the incoming light (45°) at this early (the intra-pulse) phase of the interaction, the electric-field component parallel to the surface ( E y ) exhibits a strong asymmetry ( Fig. 2b–e ). Protons gain momentum in the non-target-normal direction, which is indicated by the inclusion of the trajectories of protons that finally reach highest energies (above 90% of the maximum energy E >0.9 ) into the field maps. Already at t =44 fs (~1.5 τ ) the initial asymmetry of E y has almost vanished. From this point onwards, the self-similar expansion phase of TNSA takes over (visible in the E x field map) and further drives the proton front. Because of the laminar expansion [12] in this post-pulse phase, the intermediate deflection angles are conserved, as illustrated in Fig. 2f , whereas in the intra-pulse phase, the angle grows with time. The increase of the maximum energy of protons propagating under sample angles of 6°, −1° and −5°, which is related to the maximum field integral, provides a quantitative distinction of both phases. In the intra-pulse phase and along the optimum angle of 6°, the proton energy grows significantly faster than along other angles and than in the post-pulse phase. The initial angle-dependent disparity in energy is maintained throughout the later quasi-neutral expansion phase of the sheath. The major finding is that already at t ~2 τ , about half of the final energy can be reached. It is likely that this fraction constitutes only a lower limit for the intra-pulse energy gain, as two-dimensional particle in cell simulations, at reduced density, tend to underestimate the dilution of the sheath that is responsible for the post-pulse acceleration phase. Figure 2: Modelling the intra-pulse acceleration. ( a ) False-colour image (logarithmic scale) of the angularly resolved electron energy distribution at the target rear side, at the time the peak of the laser pulse reaches the front side ( t =0). The components of the spatial distribution of the electric field amplitude in target normal direction ( E x ), and parallel to the target surfaces ( E y ), are plotted in ( b ) and ( c ) for t =0, and in ( d ) and ( e ) for t =44 fs, respectively. The field distributions are normalized using the maximum field values of The edge size of the boxes ( b – e ) corresponds to 18 μm. The trajectories of protons reaching more than 90% of the maximum energy ( E >0.9 ) are overlaid in black. ( f ) For these protons, the increase of the deflection angle α cent with time is shown in green, together with the evolution of the maximum energy of protons emitted under sample angles α of 6° (blue), −1° (black) and −5° (red). For illustration of the timescale, the laser pulse profile is given by the red shaded region and the black gaussian-shaped curve. For the duration of the laser pulse τ , the asymmetry of the electron distribution translates into a non-target-normal emission of energetic protons that can be detected experimentally. Full size image To emphasize the relevance of the directed intra-pulse acceleration, averaged trajectories of protons reaching (0.6−0.8) E max are overlaid with the experimental spectrum in Fig. 1b . It turns out that these sample protons, finally observed under angles deviating from the optimum, gained significant energy under initially optimum angles ( α >0), and only later, got deflected owing to variations in the lateral position in the expanding plasma. Summarizing so far, the detection of prominent non-target-normal emission of energetic protons may serve as a diagnostic for an efficient intra-pulse acceleration. However, an expanding sheath can inherit geometrical properties of the target rear surface such as, for example, deformations caused by nanosecond prepulse-driven hydrodynamic shocks [4] , [13] , [14] . Thus, to unambiguously demonstrate the relevance of the intra-pulse acceleration phase, a test experiment only relying on properties of the ultrashort laser pulse itself has been designed. Proton steering by engineered laser pulse front tilts In the test experiment, sketched in Fig. 3 , the foil is irradiated under normal incidence. Additionally, a small angular chirp, being equivalent to a pulse front tilt of the ultrashort laser pulse [15] , is introduced (for details, see Methods ). It has recently been shown [16] that a small pulse front tilt directly influences the pointing of electrons accelerated in an underdense plasma. Here the pulse front tilt is used to cause a spatiotemporal asymmetry in the laser plasma interaction that is restricted to the coherent ultrashort pulse. It does not apply to the incoherent nanosecond prepulse level originating from amplified spontaneous emission. Because different laser wavelength components exhibit different incident angles on the focussing optics, the angular chirp further causes a spatial chirp in the focal plane, which leads to the oval focal spot in Fig. 3b confirming the setting. 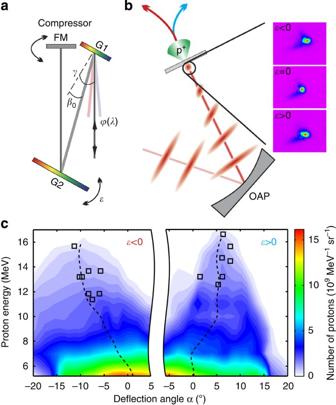Figure 3: Set-up and results of the test experiment. (a) Grating compressor consisting of the gratings G1 and G2 and the folding mirror FM. The incidence angle γ and the diffraction angleβ0are necessary to calculate the angular chirpd/dλ(equivalent to pulse front tilt) generated by a slight tilt of G2 by the angle(seeMethods). (b) The tilted intensity envelope is focussed by the off-axis parabola (OAP) under normal incidence onto a 2-μm thick Ti-foil target. The spatial chirp in the focal plane caused by the angular chirp results in horizontally enlarged focal spots, as displayed in the three images for the according settings of. (c) On the basis of the change of sign in the designed pulse front tilt, the most energetic protons are deflected away from the target normal, as it is shown by two samples of reconstructed angular proton spectra for>0 and<0. Black squares represent the scattering of the deflection angle of the most energetic protons for the full series of shots. The dashed line follows the centroid of the angular distribution. Figure 3: Set-up and results of the test experiment. ( a ) Grating compressor consisting of the gratings G1 and G2 and the folding mirror FM. The incidence angle γ and the diffraction angle β 0 are necessary to calculate the angular chirp d /dλ (equivalent to pulse front tilt) generated by a slight tilt of G2 by the angle (see Methods ). ( b ) The tilted intensity envelope is focussed by the off-axis parabola (OAP) under normal incidence onto a 2-μm thick Ti-foil target. The spatial chirp in the focal plane caused by the angular chirp results in horizontally enlarged focal spots, as displayed in the three images for the according settings of . ( c ) On the basis of the change of sign in the designed pulse front tilt, the most energetic protons are deflected away from the target normal, as it is shown by two samples of reconstructed angular proton spectra for >0 and <0. Black squares represent the scattering of the deflection angle of the most energetic protons for the full series of shots. The dashed line follows the centroid of the angular distribution. Full size image The energy-resolved proton emission pattern was recorded with RCF stacks and stacked scintillators with online camera readout for two opposite angular chirp settings. Proton spectra reconstructed from exemplarily chosen stacks are displayed in Fig. 3c . As in the previous experiment at oblique laser incidence, the highest proton energies are observed under angles of up to 10°. Clearly, the sign of the deflection from target normal only depends on the orientation of the pulse front tilt, a quantity linked to the main pulse and therefore independent from pre-pulse-induced target deformations. This observation, which could be reproduced also for thicker targets (3 μm thick), confirms that protons are significantly accelerated in the intra-pulse phase of ultrashort pulse lasers, and, additionally, provides a novel method for active fine-steering of the energetic proton bunch. Directed electron generation by the v×B force The given interpretation of both experiments further relies on the assumption that laser energy is converted into hot electrons in a directed way, as introduced in Fig. 2a . Such behaviour can be expected in the presence of a small scale length preplasma for relativistic laser intensities, where the v × B force dominates, and consistent behaviour was observed in earlier experiments detecting Cerenkov or coherent transition radiation at the target rear side [17] , [18] . The v × B dominated absorption mechanism further implies that the performance of the proton acceleration process is mostly independent of the angle of incidence of the laser beam on the foil and of the orientation of its linear polarization. Such dependencies have however been reported at lower intensities and extreme pulse contrast where the Brunel heating mechanism is dominant [19] , [20] . Relative maximum proton energies are presented in Fig. 4 for different angles of incidence as a function of the effective target thickness d eff ( d eff = d foil for δ =0° and for δ =45°) for the present interaction conditions. The decrease in intensity by for the case of δ =45° has been taken into account by the proper choice of the laser energy for the normalization shots. In conclusion, the target thickness scan reveals no dependence on the angle of incidence, which compares well with recent results [21] . Independently, the laser polarization was varied with a thin half-wave plate close to the focussing optics ( Fig. 1 ). Apart from a slight enhancement of about 10% for p -polarization with respect to s -polarization under oblique incidence, no dependence of the proton acceleration on laser polarization orientation was observed. Both findings support the v × B dominated laser light conversion into directed electrons. 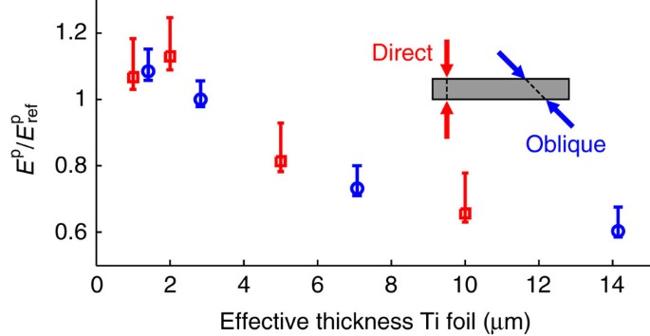Figure 4: Relative maximum proton energies for different angles of incidence. For shots under oblique incidence, the relative maximum proton energies are plotted as a function of the effective foil thicknessIn the case of direct (normal) incidencedeff=dfoilwas used. Maximum proton energiesEpare normalized to those obtained for a reproducible reference configuration(2-μm thick titanium foil atδ=45°,p-polarization). The error bars reflect the standard deviation for averaging multiple shots, and include systematic errors caused by the RCF measurement. Figure 4: Relative maximum proton energies for different angles of incidence. For shots under oblique incidence, the relative maximum proton energies are plotted as a function of the effective foil thickness In the case of direct (normal) incidence d eff = d foil was used. Maximum proton energies E p are normalized to those obtained for a reproducible reference configuration (2-μm thick titanium foil at δ =45°, p -polarization). The error bars reflect the standard deviation for averaging multiple shots, and include systematic errors caused by the RCF measurement. Full size image The experimental identification of the relevance of the intra-pulse acceleration phase for the energy gain of protons in laser plasma acceleration provides important new insight into the understanding of TNSA in the ultrashort pulse regime. Where up to only recently, the self-similar expansion of the electron sheath has been considered to be the most relevant process; for ultrashort and ultra-intense pulses, the influence of the initial state of the isothermal expansion phase [8] becomes dominant. This state is characterized by a time-independent electric field distribution and not only matches the quasi-static conditions of the intra-pulse phase but also matches the model by Schreiber et al . [5] In this model, maximum proton energies are obtained from the integration of the equation of motion in the electro-static potential that originates from a laterally confined surface charge on the target rear side for the duration of the laser pulse. An extrapolation of this approach to ultrashort pulse durations, implying that the particle remains in the vicinity of the surface charge, improves the scaling of the maximum proton energies with laser intensity from a square-root dependence to near-linear [4] . A similar behaviour can be derived from the time-limited fluid model by Mora et al . [8] for ultrashort laser pulses [22] . In practice, this novel regime motivates the application of the upcoming class of ultra-compact petawatt lasers with high pulse repetition rate. If the scaling holds true for the envisaged increase in intensities, the presently achieved proton energy level suggests that proton pulses with energies >100 MeV, mandatory for applications such as ion beam cancer therapy [23] , could be in reach. Already now, the simplicity of the approach, only requiring robust micron-thick metal targets allowed for systematic radiobiological studies [24] at the quality level of dose control of conventional proton sources. Intra-pulse acceleration exhibits the same favourable near-linear intensity scaling, as it is predicted for the far more demanding regime of radiation pressure acceleration of protons from ultrathin linear density matched foils [25] , [26] , [27] . A prepared composition of source layers on the back of the foil could lead to well-defined starting conditions of the fast acceleration and thus to monoenergetic features [28] , [29] . With the use of two independent laser pulses, a staged approach based on an intra-pulse injector and a longer plasma post-acceleration could improve energy and control of laser accelerated proton beams in the future. Laser The 150 TW Ti:sapphire laser Draco operated by Helmholtz–Zentrum Dresden–Rossendorf [4] provides pulses with τ =30 fs duration (full-width at half-maximum (FWHM), bandwidth ~60 nm, central wavelength 800 nm) and up to 4 J energy on target. For the present experiment, the 10-cm diameter beam was focussed with an F/2.5 off-axis parabolic mirror to a spot size of about 3 μm FWHM. Making use of a deformable mirror for the far-field optimization, about 80% of the energy of 2.3 J on target is contained in the central spot leading to a peak intensity of 8×10 20 W cm −2 . The spectral phase of the pulse is monitored with a spectral phase interferometer for direct electric field reconstruction and optimized in a closed loop using a DAZZLER (Fastlite). The temporal pulse contrast, achieved by the introduction of saturable absorbers into the laser chain, is measured ( Supplementary Fig. S2 ) with a high dynamic range third-order autocorrelator SEQUOIA (Amplitude Technologies). The controlled angular chirp d /dλ in the test experiment is introduced by a slight rotation of one of the compressor gratings around the axis parallel to its grooves by =±0.03° ( Fig. 3 ). Pointing is corrected for by turning the folding mirror accordingly. Given the incidence angle γ , the diffraction angle β 0 , and the groove spacing s , the angular chirp reads ±1.7 μrad nm −1 . Its value has been verified using an interferometric field autocorrelator with spatial inversion [30] . Potential changes in the group delay dispersion are compensated for by the usual optimzation procedures for grating distance and spectral phase control loops. Changes in the pulse contrast are ruled out by third-order autocorrelation measurements. In addition to the main pulse coherent pre-pulses on the picosecond timescale may also be affected by an angular chirp. Yet, their contribution to a shock-induced potentially asymmetric deformation of the target rear surface can be safely neglected for the given experimental conditions. Numerical modelling The 2D3 V particle in cell code PICLS is employed to simulate the interaction of a Gaussian-shaped laser pulse with 30 fs duration and linear p -polarization with a solid target at an angle of incidence of 45°. The target, a 1-μm thick titanium foil covered on both sides with a 30-nm thick layer of hydrogen and carbon atoms is located 35 μm from the starting edge of the simulation box. The focal spot size of 5 μm FWHM yields a peak intensity of 10 21 W cm −2 . For the realistic simulation of prepulse-induced effects like the expansion of surface layers of the foil ( Supplementary Fig. S3 ), the measured temporal profile of the laser pulse was used starting at t =−3.5 ps, where the ionization threshold is reached ( Supplementary Fig. S2 ). The simulation box consists of 19,440×8,330 cells with 55 cells per λ =800 nm and 2 ions per species and cell. The resulting electron density in the bulk is 122 n c when fully ionized. Ionization and collisions are included in the simulation. Proton detectors As the principle detector type, stacks of RCF dosimetry media mounted a few centimeters behind the target foil were used. The stacks consisted of one layer GafChromic HD and up to 15 layers of EBT films, covered with a 13-μm aluminum filter. The EBT films are absolutely dose calibrated. Besides yielding the spatial (and thus angular) distribution of the proton fluence, the RCF stacks provide a coarse energy resolution due to the energy-range relationship of the stopping power. From the depth-dose profile recorded in a single shot, spatially resolved proton spectra can be reconstructed similar to the method presented in ref. 31 . To allow for online measurements of the proton deflection angle, a stack of 0.2-mm thick scintillating screens, each of them covered with a light-tight foil, are used. The upper side surface of the stack is imaged to a camera providing an energy-selective projection of the angular distribution for each individual layer. Both techniques are routinely cross-checked with a Thomson parabola spectrometer. How to cite this article: Zeil, K. et al . Direct observation of prompt pre-thermal laser ion sheath acceleration. Nat. Commun. 3:874 doi: 10.1038/ncomms1883 (2012).